A nonspecific defensive compound evolves into a competition avoidance cue and a female sex pheromone The evolution of chemical communication and the origin of pheromones are among the most challenging issues in chemical ecology. Current theory predicts that chemical communication can arise from compounds primarily evolved for non-communicative purposes but experimental evidence showing a gradual evolution of non-informative compounds into cues and true signals is scarce. Here we report that females of the parasitic wasp Leptopilina heterotoma use the defensive compound (−)-iridomyrmecin as a semiochemical cue to avoid interference with con- and heterospecific competitors and as the main component of a species-specific sex pheromone. Although competition avoidance is mediated by (−)-iridomyrmecin alone, several structurally related minor compounds are necessary for reliable mate attraction and recognition. Our findings provide insights into the evolution of insect pheromones by demonstrating that the increasing specificity of chemical information is accompanied by an increasing complexity of the chemical messengers involved and the evolution of the chemosensory adaptations for their exploitation. Chemical senses are the oldest and most widespread in nature and chemical communication was likely the original mechanism of information transfer between individuals [1] . One major advantage of chemical communication is the enormous diversity of potential signals. To date, several thousand chemical pheromone components (chemical signals used for intraspecific communication) are known to science [2] , and using these compounds in combination results in an astounding collection of possible chemical signals. What is the origin of a chemical signal and what qualifies a certain compound to be used as a pheromone? Even considering all of the physiological and physical limitations, such as the availability of chemical precursors and biosynthetic pathways or functional signal constraints such as volatility, hundreds or thousands of different chemical compounds would be equally well suited as messengers. Thus, other factors must have a role in the evolution of such signals. Current evolutionary theory predicts that pheromones may evolve from compounds already in use for non-communicative functions [3] , [4] , [5] . For example, hormones, defensive secretions or cuticular compounds can be the basis for pheromone evolution. If these compounds, or their metabolites, are released by one individual and perceived by another individual, they might provide information about the condition of the sender. This condition can be the simple presence of the sender or, in the case of hormones, a physiological state [6] . A compound perceived in this way serves only as a cue: it supplies information without being selected for this function. If the sender benefits from the receiver’s response, chemical ritualization may alter the status of the cue into a true signal by it being selected for information transfer [3] , [7] . The use of a chemical substance for two or more purposes is well established and referred to in the literature as ‘semiochemical parsimony’ [8] . Classic examples of primarily non-communicative compounds becoming informative in intraspecific interactions are cuticular hydrocarbons (CHCs). Found on the cuticle of almost every insect, CHCs function primarily as a desiccation barrier [9] . But in addition, CHCs serve as semiochemical cues (for example, nestmate recognition in social insects) or have even evolved into signals [10] , and in some cases, the selective forces driving this process have been identified [11] , [12] , [13] . Defence compounds are also candidate chemicals that may be employed for intraspecific information transfer. To fulfil their function, they are typically produced and released in relatively large quantities and thus are often easily detectable. Consequently, defensive compounds have been found to function as alarm pheromones (for example, ref. 14 ) or even more specifically as sex pheromones [15] , [16] , [17] . However, most studies investigating multifunctional defence compounds are limited to the description of the multiple functions of the compounds but do not address the ecological framework that might have favoured their evolution. In particular, it is unclear how an increase in specificity and information reliability is achieved when defence compounds evolve into chemical cues or signals, because the same defence chemicals are often used by several species [18] . One way the specificity and reliability of the information could increase is via species-specific alterations of the chemical messengers. Such alterations could include the presence and relative proportion of other compounds in the blend. However, to the best of our knowledge, experimental evidence for this type of signal evolution is missing. Leptopilina heterotoma is a solitary larval parasitoid of Drosophilid flies, including Drosophila melanogaster [19] , [20] . Owing to the model status of its host, Leptopilina has been intensively studied during the past years (as reviewed in Fleury et al. [21] ). Recently we have shown that females and males of L. heterotoma produce iridomyrmecins in a cephalic gland and that the wasps use it as a repellent against insect predators [22] . Furthermore, it is known that females of L. heterotoma are able to distinguish between host patches with and without conspecifics, based on olfactory cues only [23] . Iridomyrmecin is the major volatile compound produced by L. heterotoma and therefore it is a likely candidate to serve as a competition avoidance cue for female L. heterotoma . Males and females of L. heterotoma use different stereoisomers of iridomyrmecin for defence. While females produce (−)-iridomyrmecin and, in much smaller quantities (+)-isoiridomyrmecin [22] , males produce only (+)-isoiridomyrmecin. This sex-specific difference and the observation that males are attracted to virgin females by olfactory signals [24] suggest that (−)-iridomyrmecin, in addition to its defensive function, might also be the female sex pheromone in L. heterotoma . In this study, we present a case of threefold semiochemical parsimony in L. heterotoma and provide evidence for the evolution of a nonspecific defensive compound into an agent mediating inter- and intraspecific competition avoidance and a species-specific female sex pheromone. This increased specificity of information is accompanied by a diversification of the chemical messengers and behavioural adaptations. Chemical analysis To identify the chemical cues and pheromone compounds mediating competition avoidance and mate finding, we extracted the wasps in dichloromethane (DCM). The extract contains iridoids and CHCs ( Fig. 1a ). We subsequently fractionated the extract into CHCs and iridoids by solid-phase extraction or size-exclusion chromatography (SEC). The iridoid fraction contained (−)-iridomyrmecin as major component ( Fig. 1b , ‘p5’) and (+)-isoiridomyrmecin (‘p6’) as a minor component. In addition, three further iridoids (‘p1’, ‘p2’, ‘p7’) were present in small amounts. 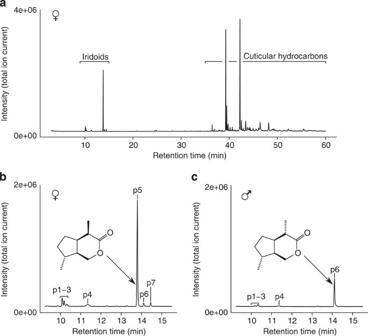Figure 1: Chemical compounds produced byL. heterotoma. Total ion current chromatograms of (a)L. heterotomafemale extract and the iridoid fraction of (b) female and (c) male extract. Compound p5 is (−)-iridomyrmecin and p6 is (+)-isoiridomyrmecin. The inserts in (b) and (c) show their structure and absolute configuration. Compounds p1 and p2 were tentatively identified as iridodials; p7 was tentatively identified as a third iridomyrmecin. p3 and p4 were behaviourally inactive and thus not identified. Figure 1: Chemical compounds produced by L. heterotoma . Total ion current chromatograms of ( a ) L. heterotoma female extract and the iridoid fraction of ( b ) female and ( c ) male extract. Compound p5 is (−)-iridomyrmecin and p6 is (+)-isoiridomyrmecin. The inserts in ( b ) and ( c ) show their structure and absolute configuration. Compounds p1 and p2 were tentatively identified as iridodials; p7 was tentatively identified as a third iridomyrmecin. p3 and p4 were behaviourally inactive and thus not identified. Full size image Mass spectra of p1 and p2 were very similar to a published mass spectrum of iridodial ( Supplementary Fig. S1a–c , ref. 25 ) suggesting that p1 and p2 are stereoisomers of iridodial. As synthetic references for iridodial were not available, we produced them by catalytic hydrogenation of (epi-)/chrysomelidial ( Supplementary Fig. S2 ) extracted from Phaedon cochleariae larvae. Two iridodials formed by hydrogenation of (epi-)/chrysomelidial showed mass spectra identical to those of p1 and p2, respectively ( Supplementary Fig. S1 ). Additionally, these iridodials co-eluted with p1 and p2 on a non-polar GC-column ( Supplementary Fig. S3 ). One of the (epi-)/chrysomelidial-derived iridodials co-eluted with p2 also on the BetaDEX 225 column ( Supplementary Fig. S4 ). We conclude from these results that p1 and p2 are iridodials. We suggest that p2 is identical to one of the (epi-)/chrysomelidial-derived iridodials, whereas p1 is likely the enantiomer of one of the other iridodials formed by hydrogenation of (epi-)/chrysomelidial. Peak p7 showed a mass spectrum similar to (−)-iridomyrmecin ( Supplementary Fig. S5a,b ) suggesting that p7 is another stereoisomer of iridomyrmecin. Mass spectra of trans-fused stereoisomers of iridomyrmecin show different mass spectra (m/z 95 is always smaller than m/z 81, Supplementary Fig. S5c , ref. 26 ) and we thus excluded the presence of these compounds. From the eight possible cis-fused stereoisomers of iridomyrmecin we excluded (+)- and (−)-iridomyrmecin and (+)- and (−)-isoiridomyrmecin because of differing retention times compared with authentic standards. Thus, four possible cis-fused iridomyrmecin stereoisomers remained as possible structures for p7. Although, those were not available as pure synthetic references, p7 co-eluted with a minor impurity in the synthetic sample of (−)-iridomyrmecin on both the non-polar BPX-5 ( Supplementary Fig. S6 ) and the Gamma DEX 120 column ( Supplementary Fig. S7 ). This impurity shows the same mass spectrum as p7 ( Supplementary Fig. S5a,d ). We therefore conclude that p7 is the same compound as the impurity in the synthetic sample. The way we synthesized (−)-iridomyrmecin suggests that this impurity, and therefore p7, is either (4 R ,4a S ,7 R ,7a R )- and/or (4 S ,4a S ,7 R ,7a R )-iridomyrmecin ( J and K in Supplementary Fig. S13 ). The line of argumentation for this conclusion is provided in detail below. Two further minor compounds in the iridoid fraction (‘p3’, ‘p4’) were found to be behaviourally inactive (see below) and were thus not structurally elucidated. Unlike (−)-iridomyrmecin and (+)-isoiridomyrmecin the minor compounds in p1, p2 and p7 were not available as synthetic standards. To test their contribution to the biological activity, we isolated them from the iridoid fraction by preparative gas chromatography. The two iridodials (p1 and p2) could not be further separated and were thus tested together in the bioassays. The CHC fraction was behaviourally inactive and thus not analysed any further. We used female L. boulardi and extracts thereof to test the species-specificity of the chemical communication in L. heterotoma. Leptopilina boulardi occurs sympatrically with L. heterotoma and parasitizes he same host species [20] , [24] . Our chemical analyses revealed that females of L. boulardi produce the same iridoid compounds as L. heterotoma females, but in different ratios ( Supplementary Fig. S8–S11 ). Detailed argumentation for the identity of p7 Because of the way the authentic standards of (−)-iridomyrmecin and (+)-isoiridomyrmecin were prepared, certain minor impurities are likely to contaminate the authentic standards. Authentic standards of (−)-iridomyrmecin and (+)-isoiridomyrmecin were prepared using a highly diastereoselective synthesis. The stereochemistry in the final products is governed by the stereochemistry of the single stereocenter in the starting material. The parlay of stereochemistry from the C7 stereocenter in citronellal to the bridgehead positions (C4a and C7a) occurs during formation of the five-membered ring. This reaction is thought to occur by a concerted hetero-Diels-Alder reaction because only products with a cis ring junction have ever been observed. With a stereocenter at C7, there are two distinct transition states for the Diels-Alder reaction that have different energies ( Supplementary Fig. S12 ). The formation of the trans cis product ( A ) is presumably favourable both kinetically because of the lower energy transition state and thermodynamically because there is less steric compression compared with the alternative cis cis product ( B ). As first described by Schreiber et al. [27] , the ratio of A to B strongly favors A under both kinetic and thermodynamic conditions. Specifically, he found that the ratio of A to B at short reaction times to be about 4:1. If the reaction is allowed to continue for long reaction times, the ratio of A to B increases to >20:1. We have used this method to generate the iridoid carbon framework extensively and have never isolated B and because it forms in such small proportions with respect to A , we have not seen evidence of it in our spectral analysis. Chances are high that the cis cis diasteromer B is present in our product mixtures albeit in very small relative amounts. In contrast, there is little chance that the cis trans or trans trans isomers ( Supplementary Fig. S12 , in the box) will form because of the stereospecificity of the concerted Diels-Alder reaction. The stereochemistry of the stereocenters at C4a, C7 and C7a do not change during the remainder of the synthesis of iridomyrmecin and isoiridomyrmecin. However, the stereocenter at C4 is generated with low selectivity later in the synthesis ( Supplementary Fig. S13 ). During the hydration of C (and D ), the C4 and C3 stereocenters are formed in all possible orientations. Using silica gel chromatography, the hydrated products E and G can be separated. Because we do not detect the alternate products derived initially from B (via D ), F and H , we cannot determine whether either F and/or H is/are present as impurities in E or G . So when E and G are separately oxidized to form (−)-iridomyrmecin and (+)-isoiridomyrmecin, we cannot say whether J and/or K is/are present as very minor impurities. In summary, although the authentic standards of (−)-iridomyrmecin and (+)-isoiridomyrmecin are very pure (>99%), it is possible that two side products, J and K , formed during their synthesis. Although it is possible that one or both of these side products are present, it is very unlikely that the corresponding cis trans or trans trans isomers (derived from the intermediates in the box in Supplementary Fig. S12 ) are present. Because a very minor component (p7) of the natural blend rich in (−)-iridomyrmecin co-elutes with a very minor impurity in the authentic standard of (−)-iridomyrmecin and has an identical mass spectrum, it is likely the identity of the minor component (p7) is either J or K . When the authentic standard of (−)-iridomyrmecin is injected with the natural compounds, the minor impurity in the authentic standard co-elutes with p7 on both non-chiral ( Supplementary Fig. S6 ) and chiral columns ( Supplementary Fig. S7 ). This is consistent with the idea that p7 forms as a side product during the biosynthesis of the (−)-iridomyrmecin in the insect produced blend. One would not expect the insect to produce the enantiomer of p7 (called here ent-p7 ). This enantiomer ( ent-p7 ) would be indistinguishable from p7 on the non-chiral GC-column but not on a chiral phase GC-column. The enantiomers of J and K , ent-J and ent-K , would be expected as minor impurities in the preparation of (+)-iridomyrmecin. Therefore, one would anticipate that the minor impurity in (+)-iridomyrmecin will co-elute with p7 on the non-chiral column and not co-elute on the chiral phase column. This expected result is borne out by experiment further supporting that p7 is J and/or K . All lines of evidence support that p7 is J and/or K . Our understanding of the synthesis of (−)-iridomyrmecin implicates J and K as likely impurities in the authentic standard. Without the isolation and full characterization of the impurity, we cannot prove that J and/or K are the structures we propose but it is highly likely based on the chemistry. Competition avoidance cue Having the volatiles produced by L. heterotoma at hand, we used a y-tube olfactometer to test the hypothesis that the iridoids, particularly (−)-iridomyrmecin, mediates competition avoidance in host-searching females of L. heterotoma . In a first basic experiment, we demonstrated that mated female L. heterotoma prefer host patch odour to clean air ( Fig. 2a ). In subsequent experiments, the responding females had the choice between the odours of two host patches, one with females, one without. Females avoided the already exploited host patches, irrespective of whether conspecific ( Fig. 2b ) or heterospecific ( Fig. 2c ) females were present and preferred the host patch without wasps. Next, we replaced the living females on the host patch with an extract of L. heterotoma females. The host patch with the female extract was avoided by the females ( Fig. 2d ), but the extract was not avoided if presented without a host patch ( Fig. 2e ). The compound(s) responsible for this effect were present in the iridoid fraction of the female extract, whereas the CHC fraction was behaviourally inactive ( Fig. 2f–g ). Finally, we added synthetic (−)-iridomyrmecin and (+)-isoiridomyrmecin, respectively, to the host patch. In both cases, the responding females avoided the modified host patches and preferred the unmodified ones ( Fig. 2h,i ). 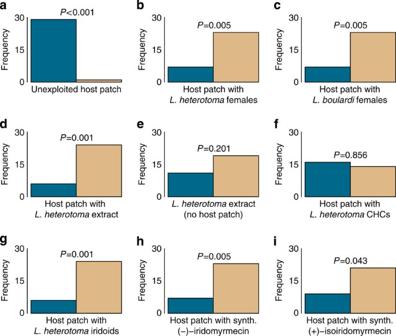Figure 2: Experiments to identify the competition avoidance cue. Frequency of decision for sample or control of matedL. heterotomafemales in a y-tube experiment when choosing between the odour of (a) a host patch and clean air, (b) an unexploited host patch and the odour of a host patch with 10 livingL. heterotomafemales, (c) an unexploited host patch and the odour of a host patch with 10 livingL. boulardifemales, (d) an unexploited host patch and a host patch with extract ofL. heterotomafemales, (e) extract ofL. heterotomafemales and clean air, (f) an unexploited host patch and a host patch with the CHCs ofL. heterotomafemales, (g) an unexploited host patch and a host patch with the iridoids ofL. heterotomafemales, (h) an unexploited host patch and a host patch with synthetic (−)-iridomyrmecin and (i) an unexploited host patch and a host patch with synthetic (+)-isoiridomyrmecin. Bar colours indicate sample (blue) and control (clean air or unexploited host patch, brown).P-values (rounded to the third decimal) are given for the two-sided binomial test. For each experimentn=30. Figure 2: Experiments to identify the competition avoidance cue. Frequency of decision for sample or control of mated L. heterotoma females in a y-tube experiment when choosing between the odour of ( a ) a host patch and clean air, ( b ) an unexploited host patch and the odour of a host patch with 10 living L. heterotoma females, ( c ) an unexploited host patch and the odour of a host patch with 10 living L. boulardi females, ( d ) an unexploited host patch and a host patch with extract of L. heterotoma females, ( e ) extract of L. heterotoma females and clean air, ( f ) an unexploited host patch and a host patch with the CHCs of L. heterotoma females, ( g ) an unexploited host patch and a host patch with the iridoids of L. heterotoma females, ( h ) an unexploited host patch and a host patch with synthetic (−)-iridomyrmecin and ( i ) an unexploited host patch and a host patch with synthetic (+)-isoiridomyrmecin. Bar colours indicate sample (blue) and control (clean air or unexploited host patch, brown). P -values (rounded to the third decimal) are given for the two-sided binomial test. For each experiment n =30. Full size image Hence, mated L. heterotoma females avoid the odour of exploited host patches. The effect is not species-specific and is mediated by (−)-iridomyrmecin and its naturally occurring epimer (+)-isoiridomyrmecin. Female sex pheromone Having demonstrated that pure (−)-iridomyrmecin mediates competition avoidance in L. heterotoma females, we asked the question whether (−)-iridomyrmecin also has a role in the attraction of males to virgin females. This hypothesis is based on the fact that (−)-iridomyrmecin is only produced by females of L. heterotoma but not by males ( Fig. 1b,c ). Again, we used a y-tube olfactometer to test this hypothesis and in a first experiment, we demonstrated that naïve L. heterotoma males were attracted by the odour of living virgin L. heterotoma females ( Fig. 3a ). Next, we replaced the living females by a solvent extract of those, which was also highly attractive to the males ( Fig. 3b ). CHCs from the female extract were not attractive to the males ( Fig. 3c ), but the iridoid fraction strongly attracted the males ( Fig. 3d ). However, pure synthetic (−)-iridomyrmecin (p5) containing its epimer (+)-isoiridomyrmecin (p6) as minor component was not attractive ( Fig. 3e ). Likewise, a blend of the minor compounds p1, p2, p3, p6 and p7 was not attractive in the bioassay ( Fig. 3f ), but adding synthetic (−)-iridomyrmecin to this mixture fully restored its attractiveness to males ( Fig. 3g ). Using (+)-iridomyrmecin instead of (−)-iridomyrmecin, however, did not restore the attractiveness ( Fig. 3h ). Males were still attracted by an iridoid fraction from which the compounds p3 and p4 had been removed by preparative GC ( Fig. 4a ). In contrast, removing either (+)-isoiridomyrmecin (p6) or the minor iridoids p1, p2 and p7, respectively, from the iridoid fraction resulted in the loss of the attractiveness ( Fig. 4b,c,d ). Doses down to 1/40 of a L. heterotoma female equivalent were attractive for L. heterotoma males in the y-tube bioassay ( Fig. 5 ). 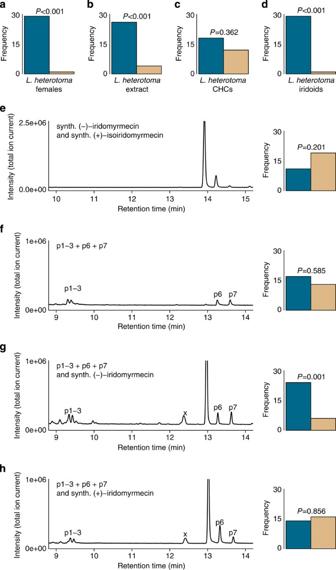Figure 3: Experiments to identify the female sex pheromone. Frequency of decision for sample or control of naïveL. heterotomamales in a y-tube experiment when choosing between the control and (a) the odour of virginL. heterotomafemales, (b) an extract ofL. heterotomafemales, (c) the CHCs or (d) the iridoid compounds from the female extract. (e–h) Total ion current chromatograms illustrating the manipulation of the iridoid fraction of the female extract and the frequency of decision in the corresponding y-tube experiment when testing the manipulated iridoid fraction against the control. Compounds p1 and p2 were tentatively identified as iridodials; p3 was behaviourally inactive and thus not identified; p6 is (+)-isoiridomyrmecin; p7 was tentatively identified as a third iridomyrmecin; x denotes contaminations.P-values (rounded to the third decimal) are given for the two-sided binomial test (a–h). Bar colours indicate sample (blue) and control (brown). For each experimentn=30. Figure 3: Experiments to identify the female sex pheromone. Frequency of decision for sample or control of naïve L. heterotoma males in a y-tube experiment when choosing between the control and ( a ) the odour of virgin L. heterotoma females, ( b ) an extract of L. heterotoma females, ( c ) the CHCs or ( d ) the iridoid compounds from the female extract. ( e – h ) Total ion current chromatograms illustrating the manipulation of the iridoid fraction of the female extract and the frequency of decision in the corresponding y-tube experiment when testing the manipulated iridoid fraction against the control. Compounds p1 and p2 were tentatively identified as iridodials; p3 was behaviourally inactive and thus not identified; p6 is (+)-isoiridomyrmecin; p7 was tentatively identified as a third iridomyrmecin; x denotes contaminations. P -values (rounded to the third decimal) are given for the two-sided binomial test ( a – h ). Bar colours indicate sample (blue) and control (brown). For each experiment n =30. 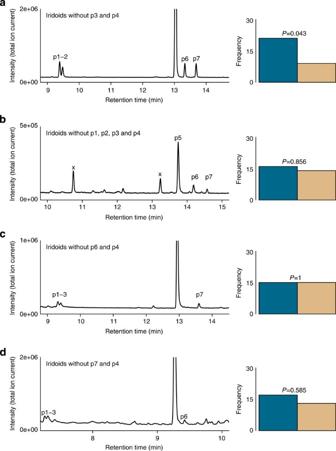Figure 4: Importance of minor components in the sex pheromone. (a–d) Total ion current chromatograms illustrating the manipulation of the iridoid fraction of theL. heterotomafemale extract and the frequency of decision for sample or control in the corresponding y-tube experiment when testing the manipulated iridoid fraction against the control. Compounds p1 and p2 were tentatively identified as iridodials; p3 and p4 were behaviourally inactive and thus not identified; p5 is (−)-iridomyrmecin; p6 is (+)-isoiridomyrmecin; p7 was tentatively identified as a third iridomyrmecin; x denotes contaminations.P-values (rounded to third decimal) are given for the two-sided binomial test. Bar colours indicate sample (blue) and control (brown). For each experimentn=30. Full size image Figure 4: Importance of minor components in the sex pheromone. ( a–d ) Total ion current chromatograms illustrating the manipulation of the iridoid fraction of the L. heterotoma female extract and the frequency of decision for sample or control in the corresponding y-tube experiment when testing the manipulated iridoid fraction against the control. Compounds p1 and p2 were tentatively identified as iridodials; p3 and p4 were behaviourally inactive and thus not identified; p5 is (−)-iridomyrmecin; p6 is (+)-isoiridomyrmecin; p7 was tentatively identified as a third iridomyrmecin; x denotes contaminations. P -values (rounded to third decimal) are given for the two-sided binomial test. Bar colours indicate sample (blue) and control (brown). For each experiment n =30. 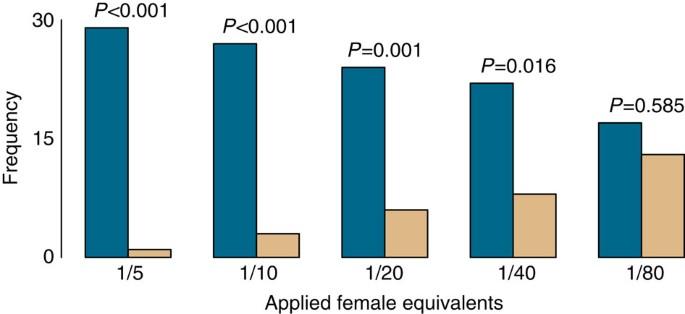Figure 5: Dose-response experiments for the sex pheromone. Frequency of decision for sample or control of naïveL. heterotomamales in a y-tube experiment when choosing between the odour of 1/5 to 1/80 female equivalent of virginL. heterotomafemale extract and the control. Bar colours indicate female extract (blue) and control (brown).P-values (rounded to third decimal) are given for the two-sided binomial test. For each experimentn=30. Full size image Figure 5: Dose-response experiments for the sex pheromone. Frequency of decision for sample or control of naïve L. heterotoma males in a y-tube experiment when choosing between the odour of 1/5 to 1/80 female equivalent of virgin L. heterotoma female extract and the control. Bar colours indicate female extract (blue) and control (brown). P -values (rounded to third decimal) are given for the two-sided binomial test. For each experiment n =30. Full size image We therefore conclude, that (−)-iridomyrmecin is the major component of the female sex pheromone in L. heterotoma and is perceived enantiospecifically. However, (+)-isoiridomyrmecin (p6), the two iridodials (p1, p2), as well as the third iridomyrmecin (p7) are also essential for bioactivity. Nonetheless, mate attraction in L. heterotoma is not species-specific, as males were also attracted by an extract of L. boulardi females ( Fig. 6a ). We therefore did an additional experiment to test whether the males discriminate between species at close range and observed the courtship behaviour (wing fanning) of L. heterotoma males towards filter paper discs impregnated with the test compounds. The duration of male wing fanning differed significantly between the test groups (Kruskal–Wallis test, H =30.4, DF=3, P <0.001). Post hoc tests indicated that males of L. heterotoma engaged in wing fanning behaviour significantly longer when exposed to paper discs treated with the iridoid fraction from conspecific females than to those treated with the iridoids from L. boulardi females, synthetic (−)-iridomyrmecin or the pure solvent ( Fig. 6b , see Supplementary Table S1 for P -values). 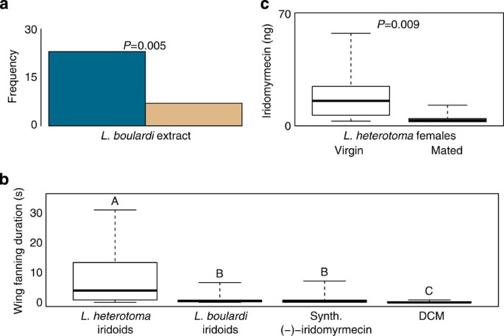Figure 6: Species-specificity and released amounts of the sex pheromone. (a) Frequency of decision for sample or control of naïveL. heterotomamales in a y-tube experiment when choosing between the control (brown bar) and the extract of virginL. boulardifemales (blue bar). TheP-value (rounded to third decimal) is given for the two-sided binomial test;n=30. (b) Box-and-whisker plots showing median (horizontal line), interquartile range (box) and maximum/minimum range (whiskers) of the duration (s) of the courtship behaviour (wing fanning) that naïveL. heterotomamales displayed towards the iridoid fraction of an extract of females ofL. heterotomaandL. boulardi, respectively, synthetic (−)-iridomyrmecin and DCM. Different capital letters above box-and-whisker-plots indicate a significant difference between these plots, cases that do not share at least one letter differ significantly (Kruskal–Wallis test followed by pairwise Mann–WhitneyU-tests with Bonferroni–Holm correction,P<0.05). For each experimentn=12. (c) Box-and-whisker plots showing median (horizontal line), interquartile range (box) and maximum/minimum range (whiskers) of the amount (ng) of iridomyrmecins released by virgin and mated females ofL. heterotoma. TheP-value (rounded to third decimal) is given for the Mann–WhitneyU-test;n=13. Figure 6: Species-specificity and released amounts of the sex pheromone. ( a ) Frequency of decision for sample or control of naïve L. heterotoma males in a y-tube experiment when choosing between the control (brown bar) and the extract of virgin L. boulardi females (blue bar). The P -value (rounded to third decimal) is given for the two-sided binomial test; n =30. ( b ) Box-and-whisker plots showing median (horizontal line), interquartile range (box) and maximum/minimum range (whiskers) of the duration (s) of the courtship behaviour (wing fanning) that naïve L. heterotoma males displayed towards the iridoid fraction of an extract of females of L. heterotoma and L. boulardi , respectively, synthetic (−)-iridomyrmecin and DCM. Different capital letters above box-and-whisker-plots indicate a significant difference between these plots, cases that do not share at least one letter differ significantly (Kruskal–Wallis test followed by pairwise Mann–Whitney U -tests with Bonferroni–Holm correction, P <0.05). For each experiment n =12. ( c ) Box-and-whisker plots showing median (horizontal line), interquartile range (box) and maximum/minimum range (whiskers) of the amount (ng) of iridomyrmecins released by virgin and mated females of L. heterotoma . The P -value (rounded to third decimal) is given for the Mann–Whitney U -test; n =13. Full size image This shows that in contrast to mate attraction, mate recognition in L. heterotoma is species-specific. This specificity is attributed to the particular blend of iridoid compounds and not to differences in the composition of the CHCs. Headspace analysis In the last experiment, we used headspace collections and GC–MS analyses to measure the amount of (−)-iridomyrmecin released by females of L. heterotoma in a non-defensive context. Virgin females released a significantly higher amount of (−)-iridomyrmecin than mated females (Mann–Whitney U -test, W =136, P =0.009) ( Fig. 6c ). Although the amount released by virgin females was much higher than in mated females, mated females still released (−)-iridomyrmecin. Our data clearly demonstrate that (−)-iridomyrmecin is not only a defensive agent in L. heterotoma but also serves as competition avoidance cue for host-searching females and as the major component of the female sex pheromone. (−)-iridomyrmecin is being used at three different levels of information transfer. As a defensive agent, it is not to be considered communicative. In competition avoidance, it serves as either cue or signal and as major component of the sex pheromone, (−)-iridomyrmecin is part of a true signal. This is exactly what current models on pheromone evolution predict: a primarily non-communicative compound may be utilized as a cue by eavesdroppers and, at the next stage, chemical ritualization may then transform the cue into a signal [3] , [4] , [5] . The hypothetical stages of this evolutionary scenario are illustrated in Fig. 7 and discussed in detail below. 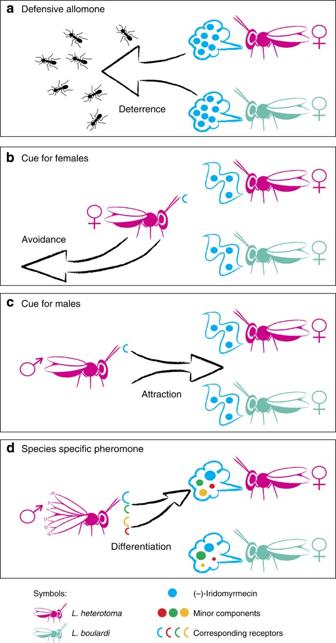Figure 7: Pheromone evolution inLeptopilina. Hypothetical stages for the gradual evolution of (−)-iridomyrmecin from a defensive compound via a semiochemical cue to a female sex pheromone inLeptopilina heterotomaas suggested by our experimental data. (a) (−)-iridomyrmecin is used as a defensive compound by females ofL. heterotomaandL. boulardi. (b) (−)-iridomyrmecin is leaking from the reservoir in small amounts in non-defensive contexts. Females ofL. heterotomause (−)-iridomyrmecin as a semiochemical cue to avoid competition with con- and heterospecific females. (c) Males ofL. heterotomause (−)-iridomyrmecin as a semiochemical cue to locate females. At this ancestral stage, males are not yet able to discriminate between the species based on the chemical cue. (d) Chemical ritualization turned the cue into a signal. (−)-iridomyrmecin and minor components are actively released by virgin females. The relative composition of (−)-iridomyrmecin and the minor components increases the reliability of the signal and creates a species-specific signal. Males ofL. heterotomadiscriminate between species and show courtship behaviour only towards conspecific females. Figure 7: Pheromone evolution in Leptopilina . Hypothetical stages for the gradual evolution of (−)-iridomyrmecin from a defensive compound via a semiochemical cue to a female sex pheromone in Leptopilina heterotoma as suggested by our experimental data. ( a ) (−)-iridomyrmecin is used as a defensive compound by females of L. heterotoma and L. boulardi . ( b ) (−)-iridomyrmecin is leaking from the reservoir in small amounts in non-defensive contexts. Females of L. heterotoma use (−)-iridomyrmecin as a semiochemical cue to avoid competition with con- and heterospecific females. ( c ) Males of L. heterotoma use (−)-iridomyrmecin as a semiochemical cue to locate females. At this ancestral stage, males are not yet able to discriminate between the species based on the chemical cue. ( d ) Chemical ritualization turned the cue into a signal. (−)-iridomyrmecin and minor components are actively released by virgin females. The relative composition of (−)-iridomyrmecin and the minor components increases the reliability of the signal and creates a species-specific signal. Males of L. heterotoma discriminate between species and show courtship behaviour only towards conspecific females. Full size image Stage one of the hypothetical scenario is the use of a certain compound for a non-communicative purpose, in the case of L. heterotoma for defence ( Fig. 7a ). Leptopilina heterotoma uses (−)-iridomyrmecin and (+)-isoiridomyrmecin as major component of their defensive secretions [22] . Actually, all stereoisomers of iridomyrmecin found in nature are effective repellents against ants and spiders [22] , [28] , [29] and thus probably against a broad range of insect predators. This suggests a conserved perception mechanism for this class of chemicals in insects, which might have been a preadaptation for the evolution of a communicative function. Apart from this, the volatility of (−)-iridomyrmecin and the fact that it is constantly available for perception from Leptopilina females ( Fig. 6c ) might have favoured this compound as a good candidate for cue or pheromone evolution. At stage two, the compound becomes a semiochemical cue. In our experiments, females foraging for hosts preferred non-exploited host patches over host patches already being exploited by conspecific or heterospecific females ( Fig. 7b ). This competition avoidance can be elicited by treating a non-exploited host patch with (−)-iridomyrmecin alone ( Fig. 2h ). (−)-iridomyrmecin can be perceived by several insects (for example, ants) [22] that have probably not been under selection to detect it. Likewise, the first eavesdropping females might have perceived (−)-iridomyrmecin without prior selection and thus could have used it as a cue. Our experiments suggest, however, that females additionally evolved a context-specific behaviour: (−)-iridomyrmecin triggers competition avoidance only when females perceive the cue with a background of host patch odour ( Fig. 2d,e ). This corroborates recent studies that have highlighted the importance of background odours for the chemical orientation of many insects in complex environments (as reviewed by Schröder and Hilker [30] ) and shows furthermore, that the avoidance behaviour of L. heterotoma females is not simply due to the repellent property of (−)-iridomyrmecin, but is indeed context-specific. We suggest that L. heterotoma females have also evolved a highly sensitive receptor, allowing them to reliably perceive even small amounts of iridomyrmecin and thus spot competitors. At the stage of competition avoidance, (−)-iridomyrmecin is at least a semiochemical cue for the females, but it could also already be a signal. A cue has not evolved to transfer information and does not essentially benefit the sender. For something to be a signal, both the emission and the response need to have evolved [31] . In our scenario, the receiver definitely benefits when favouring the unoccupied host patch over the occupied one: the sending females might already have started exploiting the resource and in L. heterotoma , earlier laid eggs have greater chances of success in cases of superparasitism [32] . On the other hand, females in an only partially exploited host patch would benefit if other host-searching females were to avoid this patch. They could then claim the remaining resources without competition. We do not know whether the females on the host patch release iridomyrmecin actively or inactively and the responding females might also behave differently if there is no unexploited host patch to choose alternatively. We can therefore not finally conclude whether the avoidance behaviour is mediated by a cue or a signal, most likely it is an intermediate evolutionary stage. In any case, in its role as competition avoidance semiochemical, (−)-iridomyrmecin gained increased specificity (compared with its use as defensive agent) through behavioural adaptations on the receiver’s side, making (−)-iridomyrmecin at least a cue. Furthermore, the competition avoidance is mediated across species’ borders. Leptopilina heterotoma females not only avoid conspecific competitors, but also heterospecific ones ( L. boulardi in this study, L. clavipes in Janssen et al. [23] ). These results are consistent with the fact that all three species occur sympatrically in Western Europe and share the same hosts [20] , [33] . Although there has been selection increasing the specificity of the cue/signal, there has been no selection for species-specificity in the response to the avoidance cue as responding females benefit by avoiding patches already exploited by females of either species. The same mechanism that allows females to avoid other females would allow males to find them ( Fig. 7c ). However, at this hypothetical intermediate stage, (−)-iridomyrmecin as sole cue is a rather unreliable means of finding a mate. Males need to distinguish between species and sexes to find a suitable mate. Using only (−)-iridomyrmecin as a cue might lead males to approach and court a different species that also produces (−)-iridomyrmecin (for example, L. boulardi ). However, in this situation, the females benefit from a reliable mate-finding mechanism as well. Selection is thus predicted to increase signal quality and modify the signal through chemical ritualization. In addition, during the cue stage, males that possess and leak (+)-isoiridomyrmecin instead of (−)-iridomyrmecin would benefit from not being courted by other males, whereas males that possess and leak (−)-iridomyrmecin would presumably be hampered in their own courtship by other males mistaking them for females. This could very well explain the sex-specific use of (−)-iridomyrmecin and (+)-isoiridomyrmecin in L. heterotoma . The third and last stage in the hypothetical evolutionary scenario outlined here is (−)-iridomyrmecin becoming a true pheromone ( Fig. 7d ). Our results show that (−)-iridomyrmecin is the major component of the female sex pheromone in L. heterotoma . However, contrary to its function in defence and competition avoidance, (−)-iridomyrmecin needs to be accompanied by several minor components to be effective as a sex pheromone ( Fig. 3g ), (−)-iridomyrmecin alone neither attracted males ( Fig. 3e ) nor elicited courtship ( Fig. 6b ). The minor components are (+)-isoiridomyrmecin (p6), the two iridodials (p1, p2) and the third iridomyrmecin (p7). Hence, all minor pheromone compounds are structurally closely related to (−)-iridomyrmecin and most probably originate from the same biosynthetic pathway. Subtle modifications of existing biosynthetic pathways may change the quantitative composition of established blends or give rise to novel pheromone components. This might lead to messenger diversification, increased signal specificity and even speciation (for example, refs 34 , 35 ). In the case of Leptopilina , the evolution of novel iridoid compounds allowed a diversification of the signal without hampering the original defensive function of (−)-iridomyrmecin. A second adaptation on the sender’s side is that virgin females release their sex pheromone actively ( Fig. 6c ). We interpret the additional use of several minor components and the active release as measures of signal amplification [3] to transform the former cue into a true and reliable signal. As the males are attracted only towards the complete pheromone blend, they have clearly adapted as well. Moreover, not only do they react to the minor components, but they also discriminate between enantiomers of iridomyrmecin. ( Fig. 3g,h ). The fact that 1/40 of a female equivalent (containing ~8 ng of (−)-iridomyrmecin) was still attractive in the y-tube assays demonstrates the high sensitivity of the olfactory receptors and the high degree of adaptation by males to the signal. The increased complexity and specificity of the sex pheromone compared with the hypothetically preceding much simpler cue illustrates the chemical ritualization necessary for the evolution of highly specific signals [3] . At the level of mate attraction, males are attracted by L. heterotoma as well as L. boulardi females ( Figs 3a and 6a ), only at close range do they discriminate conspecific and heterospecific females ( Fig. 6b ). Leptopilina heterotoma males may be attracted towards L. boulardi females, but they will discriminate con- and heterospecific females during courtship. Our results show that this species-specificity is mediated by the iridoid compounds and unlike in other parasitic wasps [36] , CHCs are not required for species recognition. As both species produce the same iridoid compounds but in different ratios, we think that these quantitative differences are responsible for species recognition and can only be reliably detected at close range. Future selection processes might favour the evolution of a long range discrimination mechanism for the males. The present study sheds new light on the chemical communication of insects by demonstrating how communicative semiochemicals evolve. Our data show the pre-adaptations that make defence chemicals likely candidates to become informative: owing to their primary function, they are available and perceivable. However, physiological adaptations are necessary on both the sender’s and the receiver’s side to fulfil the increasing demands with respect to specificity and reliability when defence chemicals evolve into cues and signals. The Leptopilina wasps studied here demonstrate that diversification of the chemical messengers and chemosensory adaptation to the modified information are a possible way for reliable and specific information transfer. Understanding the genetic and biochemical mechanisms underlying these processes will be a challenging task for future studies. Insects We reared L. heterotoma and L. boulardi using Drosophila melanogaster as host species. Drosophila melanogaster was reared on a corn-based diet (504 ml water, 66 g sugar, 6 g baker’s yeast, 2.3 g agar, 52 g cornmeal, 1.3 ml propanoic acid, 0.8 g nipagin) and kept at 25 °C, ~75% humidity and a 16:8 hL:D cycle. For each rearing, about 30 flies (mixed sexes) were placed into a jar containing fresh fly food. After 48 h, the flies were removed and ~10 mated L. heterotoma or L. boulardi females were put into the jar. Parasitized pupae were removed from the jars a few days before emergence and put singly into 1.5 ml microcentrifuge tubes to obtain unmated and naïve wasps of known age. Extraction and fractionation of compounds We extracted wasps for 10 min in 5 μl DCM per wasp. To separate iridoid compounds from CHCs, we fractionated the extract either by solid-phase extraction as described or using SEC [13] , which proved to be the more convenient method. For fractionation by solid-phase extraction, the DCM of the sample was evaporated completely under a gentle stream of nitrogen, and the sample was then redissolved in hexane. Cyanopropyl-bonded silica gel columns (50 mg, DSC-CN, Sigma-Aldrich, Taufkirchen, Germany) were pre-conditioned by rinsing them with 2 ml each of DCM and hexane; subsequently, the sample was applied to the column and eluted successively with 0.3 ml of hexane and 0.3 ml of DCM. The concentration of the fractions was determined by GC–MS and re-adjusted to the concentration of the original extract. For fractionation using SEC, we evaporated the solvent from the extract of 60 wasps, using a stream of nitrogen, reducing the sample volume to 25 μl. We then injected the sample onto a PLgel SEC column (300 mm × 7.5 mm, particle size 5 μm, pore size 100 Å, Agilent Technologies, Waldbronn, Germany) using a Rheodyne model 7125 HPLC injector equipped with a 25 μl sample loop (Rheodyne, Cotati, CA, USA). The column was connected to an LC-20AD HPLC pump (Shimadzu Europe, Duisburg, Germany) with DCM as mobile phase at a flow rate of 1.00 ml min −1 . We collected two fractions: a fraction eluting between 6.55 min–7.30 min (SEC 1) and a fraction eluting between 7.30 min–8.40 min (SEC 2). The SEC 1 fraction contained the same compounds as the hexane fraction obtained by solid-phase extraction, the SEC 2 fraction contained the same compounds as the DCM fraction (checked by GC–MS). Figure 1a shows a total ion current chromatogram of L. heterotoma female extract and indicates how this extract was fractionated by the fractionation protocols described above. The female extract and the iridoid (DCM and SEC2) fraction thereof contain (−)-iridomyrmecin (labelled ‘p5’ in Fig. 1b ), (+)-isoiridomyrmecin (‘p6’ in Fig. 1b ) and the third stereoisomer of iridomyrmecin (‘p7’), both iridodials (‘p1’ and ‘p2’) and two unidentified compounds (‘p3’ and ‘p4’), whereas males possess only (+)-isoiridomyrmecin and traces of p1, p2, p3 and p4 ( Fig. 1c ), but no (−)-iridomyrmecin [22] . To investigate the role of compounds p1, p2, p3, p4 and p7 in the putative sex pheromone, we used preparative gas chromatography to isolate these compounds from the iridoid fraction. A Shimadzu GC-2010 gas chromatograph (Shimadzu Europe, Duisburg, Germany) equipped with a non-polar capillary column (RH5-ms, 30 m length, 0.32 mm inner diameter (i.d. ), 0.25 μm film thickness, CZT, Kriftel, Germany) connected to an automated Prep 9000 fraction collection system (Brechbühler, Schlieren, Switzerland) and a Fisons GC-8000 series A equipped with a chiral cyclodextrin GC-column (BetaDEX 225, 30 m length, 0.25 mm i.d., 0.25 μm film thickness, Sigma-Aldrich, Taufkirchen, Germany) connected to a lab-made exhaustion apparatus were used for preparative gas chromatography. Carrier gas for both gas chromatographs was helium, and was employed either at a constant velocity of 50 cm s −1 (Shimadzu) or at a constant pressure of 1.2 bar (Fisons). The oven programme for the Shimadzu GC-2010 started at 80 °C and the temperature was raised by 10 °C min −1 to 280 °C and held for 13 min. For the Fisons GC-8000, the oven programme started at 100 °C and the temperature was raised by 10 °C min −1 to 200 °C and kept there for 5 min. On both systems, we trapped the compounds of interest on 10 mg Carbotrap filters (Brechbühler, Schlieren, Switzerland) and eluted them with 80 μl DCM. To obtain a natural sample of chrysomelidial as precursor for the production of iridodials, we extracted thirty larvae (L3) of Phaedon cochleariae (Coleoptera: Chrysomelidae) with 500 μl methanol for 1 h. The larval defensive secretion of P. cochleariae contains only (3 S ,8 S )-chrysomelidial (‘chrysomelidial’) as major component and minor amounts of (3 S ,8 R )-chrysomelidial (‘epi-chrysomelidial’) [37] . Synthetic compounds Synthetic reference samples of (+)- and (−)-iridomyrmecin and (+)-isoiridomyrmecin were synthesized in a diasteroselective manner from optically pure citronellal [22] . Briefly, citronellal was first converted to nepetalactol. Conversion of nepetalactol into iridomyrmecin and isoiridomyrmecin was accomplished by ionic hydrogenation, hydroxymercuration/demercuration and silver(I) oxidation [22] . Final purification was accomplished by preparative GC on the BetaDEX 225 column as described above. Hydrogenation of (epi-)/chrysomelidial to iridodial To obtain iridodial stereoisomers as reference compounds, we subjected (epi-)/chrysomelidial to catalytic hydrogenation ( Supplementary Fig. S2 ). We added a spatula tip of a Pd/C catalyst (Sigma-Aldrich, Taufkirchen, Germany) to the methanol solution of (epi-)/chrysomelidial and exposed the mixture to a weak hydrogen flow for 2 min. To remove Pd/C from the solution, we centrifuged the sample for 2 min at 8,000 r.p.m. and then transferred the supernatant to a new vial. Chemical analysis (−)-iridomyrmecin and (+)-isoiridomyrmecin were identified in L. heterotoma in a previous study [22] . We used the same methods to identify the minor components p1, p2 and p7 as well as the iridodials obtained by hydrogenation of chrysomelidial, but instead of the BetaDEX 225 column, we used a Gamma DEX 120 column (30 m length, 0.25 mm i.d., 0.25 μm film thickness, Sigma-Aldrich, Taufkirchen, Germany) for the identification of p7. Extracts of males and females of L. boulardi were analysed (including the identification of the absolute configuration of iridomyrmecin) by GC–MS. Compounds were identified by comparing the retention time (on non-polar, polar and cyclodextrin column) and mass spectra with those of reference compounds. The same methods were used to analyse the composition of the fractions obtained by solid-phase extraction or SEC. Behavioural assays We used a y-tube olfactometer to identify the competition avoidance agent and to investigate the composition of the female sex pheromone in L. heterotoma . To test the species-specificity of the chemical stimuli, we used the sympatric species L. boulardi . The y-tube was made from glass and rested at an angle of 30°, with the two arms pointing up the slope. The tube's inner diameter was 1.5 cm, the base and arms had a length of 6 cm and 9 cm, respectively. The two arms were oriented at an angle of 45°. An air pump (Fürguth, Tannheim, Germany) pumped humidified air at a combined rate of 150 ml min −1 into the tube’s arms. The setup was illuminated from above by two neon tubes (8 W). For all tests, we applied a sample to one arm and a control to the other arm. When testing extract/fractions/compounds, we always applied 1/10 female equivalent (which equals ~30 ng iridomyrmecin [22] ) or 30 ng of the synthetic compound in 2 μl solvent (test arm) or only 2 μl solvent (control arm) to small discs of filter paper. The paper discs were allowed to dry for 1 min and then placed in the upper end of each arm. To compensate for potential side preferences inherent to the experimental setup, we alternated sample and control arm regularly and turned the y-tube after every replicate. For each y-tube run, we carefully released a single individual into the y-tube's base. The test lasted for 5 min or until the individual passed a ‘decision line’, which was marked in each arm 2 cm beyond the branching point. After every other test, the y-tube was rinsed with ethanol and water. We used each individual for only one test. In the experiments conducted to identify the competition avoidance agent, we connected an Erlenmeyer flask to each of the y-tube’s arms. Each flask contained an artificial host patch consisting of 5 g of Drosophila rearing substrate (incubated with dry yeast for 2 h at 35 °C) and 20 Drosophila larvae (L1 and L2). (Experiment 1.D is an exception to this, as we did not connect Erlenmeyer flasks to the setup, see Supplementary Table S2 .) Depending on the experiment, we put five mated females into the test arm’s Erlenmeyer flask or discs of filter paper directly into the arms. In each experiment, we tested 7–10–day-old mated L. heterotoma females. To increase the number of responding females, these were allowed to lay eggs for 1 h directly before the tests. We conducted the tests 6 h after the start of the photophase, as females then show a peak in locomotor activity [38] . Each experiment was replicated 30 times. Detailed information for all conducted experiments is given Supplementary Table S2 . In the experiments conducted to identify the female sex pheromone, Erlenmeyer flasks were used only in experiment 2.A ( Supplementary Table S2 ). In all other experiments, we placed the filter paper discs directly into the y-tube's arms. In each experiment, we tested 1–3-day-old naïve L. heterotoma males. We conducted the tests 1 to 2 h after the start of the photophase. Each experiment was replicated 30 times. Detailed information for all conducted experiments is given in Supplementary Table S2 . We tested increasingly diluted samples of L. heterotoma female extract to determine the behavioural threshold for males. We used amounts representing 1/5, 1/10, 1/20, 1/40 and 1/80 of a female equivalent (corresponding to ~60, 30, 15, 8 and 4 ng of iridomyrmecin). To investigate the species-specificity of mate recognition in L. heterotoma, we observed the courtship behaviour of L. heterotoma males towards filter paper discs impregnated with the test compounds in an arena experiment. For each experiment, a disc of filter paper (5 mm diameter) was placed on a glass plate and impregnated with the test compound (in the same concentrations as in the y-tube experiments). A naïve 1–4-day-old L. heterotoma male was placed next to the filter paper and both were covered with the lid of a glass Petri dish (6 cm diameter). The male was observed for 5 min and its location and courtship behaviour (wing fanning) recorded using the software ‘The observer XT 9’. We tested the iridoid fractions of an extract of females of L. heterotoma and L. boulardi , respectively, synthetic (-)-iridomyrmecin and DCM. Amounts were equivalent to 1/10 of one female. Each experiment was replicated 12 times. The sample sizes of the behavioural experiments were chosen to be sufficient for the corresponding statistical test. Headspace analysis To compare the amount of iridomyrmecins released by virgin and mated females, we put 10 mated 2day-old females in a 100 ml Erlenmeyer flask equipped with a gas wash bottle insert (data for virgin females were taken from ref. 22 ). Air was pumped through the flask at a rate of 60 ml min −1 . Incoming air was cleaned by an activated charcoal filter; the effluent air stream passed a thermal desorption filter filled with a combined Tenax-TA/Carboxen adsorbent material (Sigma-Aldrich, Taufkirchen, Germany). For quantification, 5 ng of methyl decanoate (dissolved in methanol) were applied to the adsorbent, and the solvent was removed before volatile sampling by purging the filter for 5 min in a stream of nitrogen at a flow rate of 60 ml min −1 . Filters were thermally desorbed (8 min at 250 °C) using a Shimadzu TD20 automated thermal desorption system connected to the Shimadzu GC–MS system, described above, and analysed with the same GC and MS settings. A calibration curve was created by analysing known amounts (1–100 ng) of synthetic (−)-iridomyrmecin that were applied to the filter together with the internal standard. The experiment was replicated 13 times. Statistical analysis Behavioural data from the y-tube experiments were tested with the two-sided binomial test. Headspace data were analysed using the Mann–Whitney U -test. Data from the arena experiment were analysed with the Kruskal–Wallis test followed by pairwise Mann–Whitney U -tests with Bonferroni–Holm correction. All statistical tests were performed using R version 2.2.1 (ref. 39 ). How to cite this article: Weiss, I. et al. A nonspecific defensive compound evolves into a competition avoidance cue and a female sex pheromone. Nat. Commun. 4:2767 doi: 10.1038/ncomms3767 (2013).